Structure and properties of complex hydride perovskite materials Perovskite materials host an incredible variety of functionalities. Although the lightest element, hydrogen, is rarely encountered in oxide perovskite lattices, it was recently observed as the hydride anion H − , substituting for the oxide anion in BaTiO 3 . Here we present a series of 30 new complex hydride perovskite-type materials, based on the non-spherical tetrahydroborate anion BH 4 − and new synthesis protocols involving rare-earth elements. Photophysical, electronic and hydrogen storage properties are discussed, along with counterintuitive trends in structural behaviour. The electronic structure is investigated theoretically with density functional theory solid-state calculations. BH 4 -specific anion dynamics are introduced to perovskites, mediating mechanisms that freeze lattice instabilities and generate supercells of up to 16 × the unit cell volume in AB (BH 4 ) 3 . In this view, homopolar hydridic di-hydrogen contacts arise as a potential tool with which to tailor crystal symmetries, thus merging concepts of molecular chemistry with ceramic-like host lattices. Furthermore, anion mixing BH 4 − ← X − ( X − =Cl − , Br − , I − ) provides a link to the known ABX 3 halides. Interest in new complex metal hydrides during the past few years was initially driven by the extreme hydrogen densities and the potential to develop efficient and safe on-board hydrogen storage [1] . Metal borohydrides have large structural flexibility and display a range of other properties such as fast-ion conduction [2] , [3] or permanent nano-porosity [4] . An Na-conducting borohydride-amide has been reported as an anti-perovskite type complex hydride [5] . Until now, metal borohydrides have been obtained by synthesis approaches that are hard to control and the often rather complex new materials have little potential for structural engineering and optimization of useful properties. Rational structure-property design is most readily accomplished in very simple and stable structure types, which are capable of accommodating a wide range of different elemental compositions. Recently, we discovered the first perovskite-type metal borohydride, KMn(BH 4 ) 3 (ref. 6 ), during thermal decomposition of K 2 Mn(BH 4 ) 4 . Indeed, metal borohydrides usually crystallize with structures closely related to isoelectronic metal oxides. For instance, the polymorphs of Ca(BH 4 ) 2 are structurally related to the different modifications of TiO 2 (ref. 7 ). Prompted by these analogies, we have undertaken extensive investigations on perovskite-type borohydrides, the essentials of which we summarize here. New facile and easily scalable synthesis strategies, using a combination of solvent-based methods and mechano-chemical addition reactions, are developed for the synthesis of homoleptic perovskite-type metal borohydrides, whereas mechano-chemical metathesis reactions using metal halides provide anion-substituted metal borohydride-halides. Lanthanide borohydrides are also prepared in this study and act as precursors for both bi- and tri-metallic luminescent perovskite-type borohydrides. Thus, metal borohydrides can be utilized as ABX 3 -type host lattices. Formability of borohydride perovskites Extensive systematic synthetic work has allowed us to successfully incorporate: A =K + , Rb + , Cs + , NH 4 + , CH 3 NH 3 + , B 12 H 12 2− ; B =Li + , Mg 2+ , Ca 2+ , Sr 2+ , Sn 2+ , Pb 2+ , Mn 2+ , Y 3+ , Ce 3+ , Eu 2+ , Yb 2+ , Gd 3+ , BH 4 − and X =BH 4 − , Cl − , Br − , I − , Rb + , Cs + into the normal and inverse ABX 3 providing two new interesting perovskite-type host lattices, AB 2+ (BH 4 ) 3 and A 2 Li B 3+ (BH 4 ) 6 . Structural dynamics on the anion site are systematically introduced to the perovskite structure type, and anion substitution, where BH 4 − is partially replaced by the heavier halides, Cl − , Br − or I − , readily occurs, contributing to a vast structural flexibility and compositional diversity. Unlike most reported bimetallic borohydrides, the new series of perovskite materials shows a good thermal stability, often to 800 K, which may be lowered depending on the desired applications outlined below, effectively making them highly interesting host frameworks. However, metal borohydrides are often hygroscopic and may form di-hydrogen bonded solid hydrates, which may release hydrogen and form oxides upon heating. Hydrogen elimination and formation of oxides may occur at elevated temperatures, for example, T >350 K. The classic formability criteria for the perovskite structure type are established for the novel compound series, revealing that metal borohydride perovskites form in the range ~0.8< t <0.95, where t is the Goldschmidt tolerance factor ( Fig. 1 ). All new materials presented here have undergone a thorough crystallographic analysis. 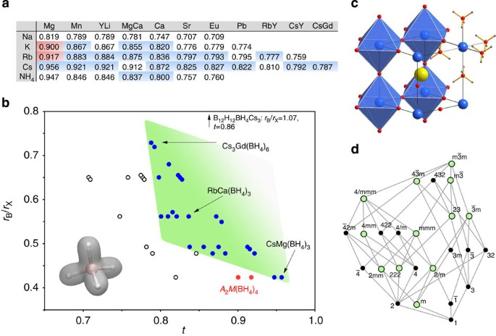Figure 1: Formability of borohydride perovskites. (a) Table of tolerance factors reportingusingrBH4~2.03 Å (ref.45). Blue fields in the table show new perovskite compounds from this study and are represented by filled blue circles inb, formability is shown as function of octahedral factor and tolerance factort. In green, the stability field of borohydride perovskites, in red the complex anion-based compoundsA2M(BH4)4are formed6. Empty circles correspond to white fields in the table and did not form the perovskite type. (c) The basicAB(BH4)3structure, highlighting the bidentate coordination mode in an ordered polymorph. (d) Sub-groups derived from the cubic aristotype, for example, SrTiO3(STO). Borohydride perovskites have been found in this study for the point group symmetries with filled green circles. Note: the compounds containing B12H122−, CH3NH3+, Ce3+and Yb2+as well as the mixed-anion variants are not listed in the table in panelabecause so far only selected systems have been tested (Supplementary Table 1). Table 1 lists the compounds most relevant to the discussion in this article and the complete list of 30 new compounds, their lattice parameters, crystal symmetries and high-temperature polymorphs is provided in Supplementary Table 1 . Figure 1: Formability of borohydride perovskites. ( a ) Table of tolerance factors reporting using r BH4 ~2.03 Å (ref. 45 ). Blue fields in the table show new perovskite compounds from this study and are represented by filled blue circles in b , formability is shown as function of octahedral factor and tolerance factor t . In green, the stability field of borohydride perovskites, in red the complex anion-based compounds A 2 M (BH 4 ) 4 are formed [6] . Empty circles correspond to white fields in the table and did not form the perovskite type. ( c ) The basic AB (BH 4 ) 3 structure, highlighting the bidentate coordination mode in an ordered polymorph. ( d ) Sub-groups derived from the cubic aristotype, for example, SrTiO 3 (STO). Borohydride perovskites have been found in this study for the point group symmetries with filled green circles. Note: the compounds containing B 12 H 12 2− , CH 3 NH 3 + , Ce 3+ and Yb 2+ as well as the mixed-anion variants are not listed in the table in panel a because so far only selected systems have been tested ( Supplementary Table 1 ). Full size image Table 1 Space group symmetries (SG), unit cell volumes and investigated properties of selected compounds. Full size table Lattice instabilities and di-hydrogen contacts Metal oxide and related perovskites usually undergo a series of temperature-induced polymorphic transformations that are of great importance for their physical properties. This sequence of structural transformations is dominated by lattice instabilities, involving phonons corresponding to both octahedral rotations and polar displacements, in addition to some degree of orbital-induced effects in most compounds. These lattice distortions are stabilized at low temperatures, when the corresponding phonons, soft modes, condense. Therefore, the perovskite structure-type evolves to higher symmetries with increasing temperature. As a consequence of the symmetry increase, inversion symmetry is usually introduced, signifying the loss of interesting polar properties, such as a simple spontaneous polarization. Hence, new ways to generate low symmetries in perovskite compounds are of interest. In the following, we show that, contrary to oxide and halide perovskites, the prototypical structural high-temperature evolution to higher symmetries does not always hold for the BH 4 -series and that di-hydrogen contacts between neighbouring BH 4 ligands appear as potential tools to tailor the symmetry. A rigorous structural investigation of KCa(BH 4 ) 3 was undertaken during a search for ferroelectric distortions. At room temperature (RT), KCa(BH 4 ) 3 is orthorhombic (BH 4 orientationally ordered) and crystallizes with the octahedral rotation pattern a 0 a 0 c + , which is characteristic of centrosymmetric tetragonal P 4/ mbm perovskites ( Supplementary Table 1 ) [8] . In the symbol a 0 a 0 c + , superscripts refer to the sense of rotation and letters to the axis of rotation. The space group symmetry P 4/ mbm, however, is lowered because of the ordering of hydrogen atoms to the polar space group Pba 2. Before the temperature-induced phase transition at 340 K, KCa(BH 4 ) 3 approaches tetragonal symmetry, following the intuitive structural evolution of perovskites ( Fig. 2 , Supplementary Fig. 1 ). The transition, however, is orthorhombic–orthorhombic, hence without symmetry increase. The changes in local structure are shown in Fig. 2c (Rietveld plots in Supplementary Figs 2–4 ). The unit cell axis c is doubled in the HT -polymorph (space group Pbn 2 1 ), introducing a further octahedral tilt ( a − a − c + ), characteristic of the orthorhombic Pnma perovskites. Space group symmetry is lowered to Pbn 2 1 , again due to hydrogen ordering. Solid-state density functional theory (DFT) calculations were performed in different symmetries for the experimentally observed KCa(BH 4 ) 3 -polymorphs, and also on the hypothetical tetragonal model, which is approached pre-transition, to determine the structural features preventing its stability. 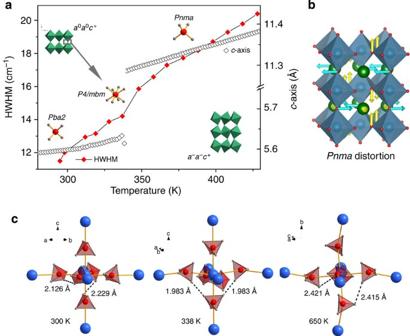Figure 2: Structural changes induced by the phase transition in KCa(BH4)3. (a) Evolution of the Raman-active symmetric bending B-H vibration illustrated by means of the half width at half maximum (HWHM), superposed by the lattice doubling inc. The jump in the bandwidth of internal vibrations is characteristic for all borohydride perovskites that undergo structural phase transitions. Structural schemes are shown for the octahedral framework ina0a0c+(RT,Pba2) anda−a−c+(HT,Pbn21) tilt patterns. Cell-doubling proceeds via intermediate BH4disorder highlighted by the grey box. (b) The lattice instability involved in the polymorphic transformation, displacement vectors are shown relative to the unstable tetragonal polymorph. (c) Local changes of the Ca(BH4)6-octahedron at different temperatures, highlighting the relevant short H···H contacts. The results are summarized in Table 2 and optimized lattice parameters can be found in Supplementary Table 2 . In Fig. 2 the minimum values for the interatomic hydrogen distances are highlighted, 2.126 and 2.415 Å in the LT and HT phases. In a fixed cell DFT optimization of the tetragonal model, this H···H distance drops to 1.983 Å. This value is considerably below the lowest values observed for borohydrides, similar to the Switendick criterion for stable hydrides [9] , 2.1 Å, which is one of the factors imposing limits on the stability of a metal hydride. An optimization in a variable cell converges to the orthorhombic lattice metric ( Table 2 ), allowing us to identify close di-hydrogen contacts between neighbouring BH 4 groups, which destabilize the tetragonal structure approached before the phase transformation. A wide range of experimental structures as well as DFT optimizations reported in the literature evidences the tendency of borohydride compounds to maximize H···H distances. Thus, assuming a repulsive nature of the homonuclear di-hydrogen contacts, we find an explanation for the unusual distortions in the high-temperature phases. In KCa(BH 4 ) 3 , the close distances are relaxed to 2.415 Å in the HT -phase by 90° flips of every second axial BH 4 group ( Fig. 2c ). The change of the octahedral tilt pattern corresponds to a very common instability in perovskites, occurring at the R -point of the Brillouin zone. The displacement generated by this instability is pointed out by arrows in Fig. 2b . In metal oxides, it involves the condensation of an octahedral rotation mode and commonly occurs in the low-temperature polymorph as a result of mode softening. In contrast, this instability is stabilized at increasing temperatures in KCa(BH 4 ) 3 , owing to a new mechanism controlled by di-hydrogen contacts and suggested by DFT calculations. This is supported by further solid-state calculations on ordered bromine-substituted variants, KCa(BH 4 ) 2 Br and KCa(BH 4 )Br 2 , which result in the stabilization of the tetragonal phase ( Supplementary Discussion ), because of the elimination of the respective short contacts by anion-substitution BH 4 − ←Br − . Structural dynamics play an important role for this mechanism. The bandwidths of Raman and infrared active B-H bending modes were monitored across the phase transition ( Fig. 2a , Supplementary Figs 5 and 6 ) and change abruptly at the critical temperature. This reflects a change in molecular B-H vibrations concurring with the lattice distortion identical in symmetry to the R -point instability, which in turn alludes to a certain degree of interaction between molecular and lattice vibrations. B-H vibrations involving critically close di-hydrogen contacts may thus be used to generate lattice distortions even at high temperatures in perovskite-type metal borohydrides. Figure 2: Structural changes induced by the phase transition in KCa(BH 4 ) 3 . ( a ) Evolution of the Raman-active symmetric bending B-H vibration illustrated by means of the half width at half maximum (HWHM), superposed by the lattice doubling in c . The jump in the bandwidth of internal vibrations is characteristic for all borohydride perovskites that undergo structural phase transitions. Structural schemes are shown for the octahedral framework in a 0 a 0 c + ( RT , Pba 2) and a − a − c + ( HT , Pbn 2 1 ) tilt patterns. Cell-doubling proceeds via intermediate BH 4 disorder highlighted by the grey box. ( b ) The lattice instability involved in the polymorphic transformation, displacement vectors are shown relative to the unstable tetragonal polymorph. ( c ) Local changes of the Ca(BH 4 ) 6 -octahedron at different temperatures, highlighting the relevant short H ··· H contacts. Full size image Table 2 DFT-optimized symmetries and calculated energies per unit cell for KCa(BH 4 ) 3 and bromine-substituted variants. Full size table These findings outlined in detail for KCa(BH 4 ) 3 are by no means restricted to specific tolerance factors but represent rather a general feature of borohydrides crystallizing with the perovskite structure. Temperature-induced lattice distortions have been discovered in various members of the AB (BH 4 ) 3 series, generating superstructures of up to 16 × unit cell volumes compared with a primitive cubic AB X 3 unit cell, of which selected examples are given in Table 1 . To our knowledge, unit cells of these dimensions have not been reported for such simple compositions. The largest superstructure is found for the commensurately modulated high-temperature polymorph HT 1-RbCa(BH 4 ) 3 , which has been stabilized at RT by Mg substitution on the B- site, shown in Fig. 3 . The structural transformation of RT -RbCa(BH 4 ) 3 into the superlattice is accompanied by a significant negative unit cell volume contraction of over Δ V / V =−1.3%, exclusively due to the modulation taking place. RbCa(BH 4 ) 3 has two other high-temperature polymorphs that evolve to higher symmetries in agreement with the common structural behaviour of perovskites ( Fig. 3d ). 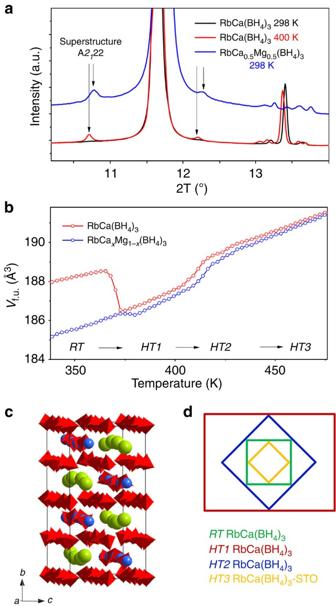Figure 3: Anomalous high-temperature behaviour of RbCa(BH4)3. (a) Superposition of X-ray diffraction patterns for RbCa(BH4)3andB-site substituted RbCa0.5Mg0.5(BH4)3showing different temperature-stability of the modulated phase. Bragg peak at 13.4°: unreacted RbBH4. (b) The large negative volume anomaly is clearly related to electrostatic repulsion generating modulation in the superstructure, which is already present at RT in the substituted compound, resulting in a much smaller volume discontinuity. (c) View approximately along thea-axis of the unit cell ofHT1-RbCa(BH4)3, showing the sinusoidal displacive modulation. (d) Schematic unit cell relationship betweenRTandHTpolymorphs of RbCa(BH4)3.HT3corresponds to a basic cubic perovskite cell. Figure 3: Anomalous high-temperature behaviour of RbCa(BH 4 ) 3 . ( a ) Superposition of X-ray diffraction patterns for RbCa(BH 4 ) 3 and B -site substituted RbCa 0.5 Mg 0.5 (BH 4 ) 3 showing different temperature-stability of the modulated phase. Bragg peak at 13.4°: unreacted RbBH 4 . ( b ) The large negative volume anomaly is clearly related to electrostatic repulsion generating modulation in the superstructure, which is already present at RT in the substituted compound, resulting in a much smaller volume discontinuity. ( c ) View approximately along the a -axis of the unit cell of HT 1-RbCa(BH 4 ) 3 , showing the sinusoidal displacive modulation. ( d ) Schematic unit cell relationship between RT and HT polymorphs of RbCa(BH 4 ) 3 . HT3 corresponds to a basic cubic perovskite cell. Full size image Systematic in-situ diffraction studies at variable temperature ( Supplementary Fig. 7 ) show that the critical temperature T c at which H ··· H interaction becomes sufficiently strong to drive a polymorphic transformation depends on the size of the A -cation, that is, T c =340, 370–410 and 515 K for KCa(BH 4 ) 3 , RbCa(BH 4 ) 3 and CsCa(BH 4 ) 3 , respectively. The hydrogen-specific interactions tend quite frequently to generate complex distortions leading to large supercells in the borohydride family of perovskites. Luminescence measurements Lanthanides form the basis of red-green-blue colours in light emitting diode (LED)-based solid-state lighting with many important applications. Eu 2+ luminescence based on the intense parity allowed transitions 4f 6 5d 1 -4f 7 is widely investigated as it is, together with Ce 3+ , the dominant activator in white light-emitting devices. A quantum yield of 75% was recently reported for the molecular compound [Eu(BH 4 ) 2 (THF) 2 ] and the absence of significant concentration quenching was attributed to the spatial separation of luminescent centres by BH 4 − (ref. 10 ). We have prepared various homoleptic lanthanide borohydrides with solvent-based methods, which act as precursors for tuneable perovskite-type host lattices. The lanthanide excited states, for example, those of Eu 2+ or Yb 2+ , are not quenched by B-H vibrations in a homoleptic BH 4 -environment, making the borohydride perovskites a new host family of phosphors. The results from spectroscopic measurements are summarized in Fig. 4 . Already neat CsEu(BH 4 ) 3 shows intense blue luminescence centred around 485 nm, 20 nm red-shifted from the precursor Eu(BH 4 ) 2 ( Supplementary Fig. 8 ). The emission intensity of Eu 2+ -activated CsCa(BH 4 ) 3 (~5 mol% Eu 2+ ) is qualitatively the same as that of bulk CsEu(BH 4 ) 3 , suggesting the effect of concentration quenching to be minimal. 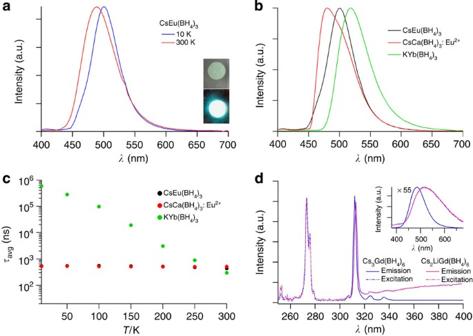Figure 4: Emission spectra and lifetimes ofREE-excited states. (a) Emission spectra (excitation at 355 nm) of CsEu(BH4)3at 10 and 300 K. A pellet is shown at room temperature, under white light and ultraviolet-excitation at 365 nm. (b) Comparison of the 10 K emission spectra (excitation at 355 nm) of bulk CsEu(BH4)3, doped CsCa(BH4)3:Eu2+and bulk KYb(BH4)3. (c) Temperature dependence of the average luminescence lifetime probed at 500 nm (excitation at 355 nm) of CsEu(BH4)3, CsCa(BH4)3:Eu2+and KYb(BH4)3. (d) Room temperature excitation (probed at 312 nm) and emission (excitation at 273 nm) spectra of Cs3Gd(BH4)6and Cs2LiGd(BH4)6. Inset: Normalized low-energy part of the emission spectra. Figure 4: Emission spectra and lifetimes of REE -excited states. ( a ) Emission spectra (excitation at 355 nm) of CsEu(BH 4 ) 3 at 10 and 300 K. A pellet is shown at room temperature, under white light and ultraviolet-excitation at 365 nm. ( b ) Comparison of the 10 K emission spectra (excitation at 355 nm) of bulk CsEu(BH 4 ) 3 , doped CsCa(BH 4 ) 3 :Eu 2+ and bulk KYb(BH 4 ) 3 . ( c ) Temperature dependence of the average luminescence lifetime probed at 500 nm (excitation at 355 nm) of CsEu(BH 4 ) 3 , CsCa(BH 4 ) 3 :Eu 2+ and KYb(BH 4 ) 3 . ( d ) Room temperature excitation (probed at 312 nm) and emission (excitation at 273 nm) spectra of Cs 3 Gd(BH 4 ) 6 and Cs 2 LiGd(BH 4 ) 6 . Inset: Normalized low-energy part of the emission spectra. Full size image Eu 2+ luminescence has also very recently been investigated in the perovskite CsCaBr 3 :Eu 2+ , serving as scintillator crystal [11] . Indeed, our results may be most readily compared with this compound as the structures are closely related. The excitation spectra both of CsCa(BH 4 ) 3 :Eu 2+ and bulk CsEu(BH 4 ) 3 are very similar and compare well to the one reported for Eu 2+ -activated CsCaBr 3 . The excitation spectrum of Eu 2+ in the borohydride extends further into the visible compared with the bromide compounds, because of a larger crystal field splitting of the 5d electron involved in the d→f transition. The emission spectrum is considerably broader in the borohydride than the bromide-based compound, which alludes to a somewhat larger geometry difference between the ground and excited states. The temperature dependence of the band position and intensity of the Eu 2+ emission was recorded between RT and 10 K, both for the doped and bulk materials, the latter being shown in Fig. 4a . Interestingly the concentration of Eu 2+ in the lattice appears to have an effect on the energy-shift with temperature. Although at RT both bulk and doped emission are centred at 485 nm, spectra obtained at 10 K ( Fig. 4b ) demonstrate a red shift of approximately 25 nm for bulk CsEu(BH 4 ) 3 , the band position being located in the green (510 nm) at 10 K. CsCa(BH 4 ) 3 :Eu 2+ , on the other hand, does not follow this temperature dependency of the emission significantly. The origin of this is attributed to the tetragonal site symmetry, the Eu 2+ centre in CsEu(BH 4 ) 3 , whereas it is cubic in the host of CsCa(BH 4 ) 3 , resulting in different thermal dilatations. In Fig. 4c the lifetimes of the excited states are presented. The exponential decay curves were described with single exponentials and are identical within experimental error for both doped and bulk materials, providing life times of approximately 500 ns for the Eu 2+ emission, which remain constant over the entire investigated temperature range. This observation shows that there is no additional non-radiative decay path activated in this temperature range, which is remarkable for a host lattice with a rich B-H vibrational structure. The reducing nature of the borohydride anion may be utilized to stabilize low oxidation states that are labile with respect to oxidation. This is the case, for example, for the divalent state of ytterbium Yb 2+ . Yb-doped crystals have been considered as potential laser crystals [12] and have attracted attention as spectral conversion materials for warm-white LEDs [13] , [14] , but limited knowledge on Yb 2+ is available when, for example, compared with Eu 2+ or Ce 3+ , because of the reducing conditions required to stabilize the divalent cation in crystals. A new stable Yb(II)-based borohydride perovskite is presented here. KYb(BH 4 ) 3 is orthorhombic and crystallizes with a commensurately modulated eightfold superlattice ( Table 1 ), whose metric has not been reported for a simple ABX 3 composition. The Yb 2+ emission is centred at 520 nm, when excited in the ultraviolet at 355 nm. The lifetime of the excited state is comparable to that of the Eu 2+ emission at RT. However, the lifetime of the Yb 2+ emission increases by three orders of magnitude between 300 and 10 K ( Fig. 4c ). A lifetime of 500 μs was determined from the decay curves at low temperatures, similar to that reported for Yb 2+ in other host materials [12] . For a parity allowed transition lifetimes in the micro-second range are quite long. Two possibilities may be that the lowest 4f 13 5d 1 state is a triplet state, which would render the transition spin-forbidden, or that the emitting state is not 4f 13 5d 1 , but 4f 13 6s 1 , which would imply Δ l =3 and hence the emission would be forbidden [12] . Investigation of trivalent lanthanide ions is more challenging and requires a host material other than, for example, CsCa(BH 4 ) 3 , adapted for divalent lanthanides. Such hosts are provided by A 3 B (BH 4 ) 6 and A 2 Li B (BH 4 ) 6 . Based on this, we have designed new B -site ordered double-perovskite materials such as Cs 3 Gd(BH 4 ) 6 , Rb 3 Ce(BH 4 ) 6 and Cs 2 LiCe(BH 4 ) 3 ( Supplementary Table 1 ), illustrating that the borohydride perovskite lattice readily accommodates Ln 3+ provided their oxidation state is stable against reduction by the BH 4 − anion, which we find to be the case for Gd 3+ or Ce 3+ , for example, but not for Eu 3+ or Sm 3+ . Luminescence spectra for Cs 3 Gd(BH 4 ) 6 and Cs 2 LiGd(BH 4 ) 6 are shown in Fig. 4d . The weaker bands occurring on the low-energy side of the sharp forbidden 6 P 7/2 → 8 S 7/2 (f-f) transition are denoted phonon-sidebands, which arise from energy-transfer to the lattice and are red-shifted by 1,400 and 2,500 cm −1 , in perfect agreement with the energies of deformation and stretching vibrations of the BH 4 molecule. The inset of Fig. 4d compares the low-energy region probed for both compounds. A broad band is visible here, which is attributed to Eu 2+ impurities contained in the reactant used in the synthesis of Gd(BH 4 ) 3 . The considerably broadened and asymmetric shape of this band can have its origin in the anomalous luminescence of Eu 2+ (ref. 15 ). Both intensity and width of this band are larger in Cs 2 LiGd(BH 4 ) 6 , likely due to a larger degree of disorder and vacancies. It is surprising that molecular B-H vibrations have no significant impact on the emission of lanthanide-excited states. Moreover, the optical properties may be tuned by halide substitution, BH 4 ←Halide, and deuterium-hydrogen exchange, 2 H←H, within the BH 4 -ligand itself. Borohydride lattices are rather ‘soft’, when compared with other hosts. This makes the emission of Ln n+ in borohydrides extremely sensitive to physical pressure, which can be relevant when applied as luminescent pressure sensors, especially in the low-pressure regime, where pressure determination remains challenging. The bulk modulus was extracted from equations of state determined for the potential hosts CsCa(BH 4 ) 3 and Cs 2 LiY(BH 4 ) 6 ( Supplementary Fig. 9 ). The softness of material is remarkably high for a perovskite (~ 26% compression at 10 GPa) and yields small bulk moduli K 0 of 27(1) and 28.3(8) GPa, respectively, similar to the larger halides but much smaller than oxides with typical values of over 150 GPa. Electronic structure The electronic structure calculated for selected compounds from the metal borohydride perovskites family shows that the compounds are wide-gap insulators of predominantly ionic nature. Covalent contributions are found for the bonding interactions between boron and hydrogen within the borohydride complex anion. This is readily seen from the partial density of states (DOSs) on the s-orbitals of hydrogen and the s- and p-orbitals of B, shown in Fig. 5a for the LT -polymorph of CsCa(BH 4 ) 3 . The relevant orbitals of both the Cs and Ca come to lie deep within the core band. Band edges are hence dominated by B-H contributions. The DOS of the materials containing Gd, Y and Eu preserves identical features as compared with the Ca-salt. Their projected DOS are summarized in Supplementary Fig. 10 . Calculated band structures ( Supplementary Fig. 11 ) show that the band gap is direct at the Γ -point for most compounds. In compliance with the detailed structural characterization of KCa(BH 4 ) 3 , the density of states and band structures were obtained for both the high- and low-temperature polymorphs of this compound to evaluate the impact of the octahedral rotations on the nature of the band gap. Interestingly, although the transition in the LT -phase is indirect, Z - Γ , because of states at the Z -point slightly higher in energy, it becomes direct, Γ - Γ , in the HT -polymorph. We recall that this transition is triggered by structural dynamics of the BH 4 , group which experiences a 90° flip in the HT -phase, and results in octahedral rotations identical in symmetry to the mentioned soft mode at the R -point. The coordinates of the symmetry point at the band gap experience a change at the valence band edge, which is exclusively occupied by boron and hydrogen states, from Γ to Z ( Supplementary Fig. 11 ). The band gap energy increases very slightly after the phase transition. In the related plumbohalide compounds, such effects have been attributed to the octahedral tilts introduced in low-symmetry polymorph [16] , [17] , whereas the tilts are not found to impact on the nature of the gap. This suggests that it is the 90° re-orientation of the borohydride anion that induces the change in band gap from indirect to direct across the transition in KCa(BH 4 ) 3 . The occupation of edge states can be modified by the introduction of elements with higher lying occupied orbitals. Remarkably, a novel caesium-lead borohydride, CsPb(BH 4 ) 3 , was synthesized ( Supplementary Table 1 ), which is the first non-molecular borohydride to contain a group IV metal, furthermore with the extreme electronegativity χ (Pb)=2.33 (refs 18 , 19 ). Lead is rare on the B -site of a perovskite, and has recently attracted considerable interest among the light-harvesting plumbohalides in modern photovoltaics [20] , [21] . Tetragonal CsPb(BH 4 ) 3 is the first semiconducting metal borohydride with an experimental band gap of ~1.5 eV determined at RT, and releases 4.3 wt% gas at ~360 K ( Supplementary Figs 12 and 13 ). The partial DOS on the Cs, Pb, B and H atoms is shown in Fig. 5b . As compared with the above-mentioned compounds, the band edges now contain a significant amount of s(Pb)-states at the valence band-edge and p(Pb)-states at the conduction band-edge, which hybridize with the ligand orbitals, hence creating covalent interactions to some extent in the octahedral Pb(BH 4 ) 3 − framework, similar to what is reported for plumbohalides [17] , [22] . Anion substitution BH 4 − ←Cl − further modifies states in the Pb X 3 − framework of substituted variants as was theoretically investigated on CsPb(BH 4 ) 2 Cl, whose DOS and band structure are summarized together with those of other compound in Supplementary Figs 10 and 11 . 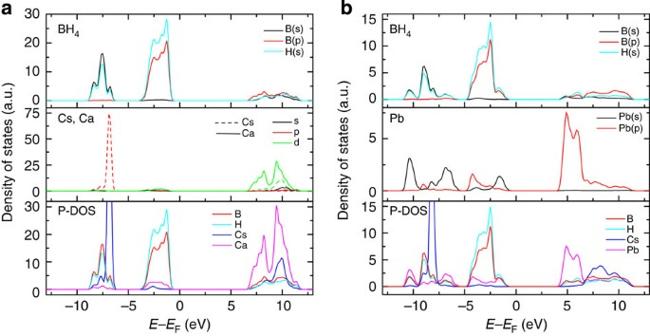Figure 5: Partial projected density of states. (a) Partial projected density of states (P-DOS) forLT-CsCa(BH4)3on the ligand orbitals (top), cations (middle) and superposed (bottom) (b) P-DOS for CsPb(BH4)3on the ligand orbitals (top),s(Pb) andp(Pb) orbitals (middle) and superposed (bottom). Figure 5: Partial projected density of states. ( a ) Partial projected density of states (P-DOS) for LT -CsCa(BH 4 ) 3 on the ligand orbitals (top), cations (middle) and superposed (bottom) ( b ) P-DOS for CsPb(BH 4 ) 3 on the ligand orbitals (top), s (Pb) and p (Pb) orbitals (middle) and superposed (bottom). Full size image Hydrogen storage properties Crystal engineering of KCa(BH 4 ) 3 (gravimetric hydrogen density ρ m =9.7 wt% H 2 ) is tempting by replacing potassium or calcium with a lighter weight cation in order to increase the gravimetric hydrogen density. However, both NaCa(BH 4 ) 3 and NaMg(BH 4 ) 3 lie outside the determined perovskite structural stability field ( Fig. 1 ). A previous report mentions high hydrogen densities in a long list of about 20 perovskite-type metal hydrides [23] , for example, NaMgH 3 , and suggested a future expansion to complex hydrides such as NaMg(BH 4 ) 3 . The smallest stable inorganic hydrogen-rich cation is NH 4 + , similar in size to K + . We have succeeded in synthesizing an ammonium borohydride perovskite NH 4 Ca(BH 4 ) 3 ( ρ m =15.7 wt% H 2 ), containing both protic and hydridic hydrogen, with short di-hydrogen bond H δ− ···H δ+ distances of 2.2 Å, thus creating a predisposition to eliminate the hydrogen molecule by thermolysis with the onset slightly above 370 K ( Fig. 6 ). NH 4 Ca(BH 4 ) 3 contains two highly disordered tetrahedral building units and can be considered the first successful stabilization of the metastable compound NH 4 BH 4 with a very high hydrogen content of ρ m =24.5 wt% H 2 . The tailoring of hydrogen storage properties by ammonia or amide has become an established approach [24] , but ammonium NH 4 + has so far not been considered. The analysis of volatile decomposition products presented in Fig. 6 shows that there is no diborane released during the decomposition of the ammonium calcium perovskite. NH 4 Ca(BH 4 ) 3 releases one molecule of hydrogen during thermolysis and transforms to a new ammonia-borane complex Ca(BH 4 ) 2 -NH 3 BH 3 ( Table 1 ), which releases additional hydrogen similar to previously reported reaction mechanisms for ammonia-borane complexes [25] , [26] . 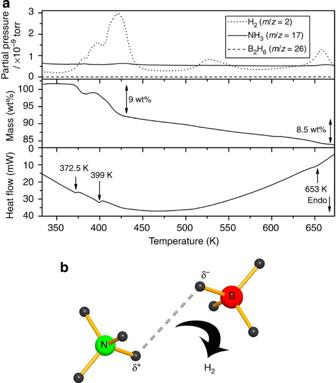Figure 6: Gas release and thermal analysis of the decomposition of NH4Ca(BH4)3. (a) Results from mass-spectrometry, thermal gravimetric analysis and differential scanning calorimetry. (b) Close hetero-nuclear di-hydrogen contact between protic hydrogen pertaining to the ammonium cation and hydridic hydrogen from the borohydride anion can facilitate hydrogen release. Figure 6: Gas release and thermal analysis of the decomposition of NH 4 Ca(BH 4 ) 3 . ( a ) Results from mass-spectrometry, thermal gravimetric analysis and differential scanning calorimetry. ( b ) Close hetero-nuclear di-hydrogen contact between protic hydrogen pertaining to the ammonium cation and hydridic hydrogen from the borohydride anion can facilitate hydrogen release. Full size image We have also prepared a hybrid organic–inorganic perovskite material, CH 3 NH 3 Ca(BH 4 ) 3 , by A -site substitution. Furthermore, an anti-perovskite structured compound Cs 3 B 12 H 12 BH 4 is discovered to form in situ during the decomposition of Cs 3 Y(BH 4 ) 6 and Cs 2 LiY(BH 4 ) 6 (Y. Sadikin, personal communication, Supplementary Fig. 14 ). This compound may be considered the first member of a new class of closo -borane perovskite-like materials and constitutes the first in-situ observation of a well-crystallized closo -borane during the decomposition of a borohydride. Higher boranes have been suggested as important decomposition intermediates of metal borohydrides during hydrogen release reactions and are often considered to be responsible for the poor reversible hydrogen storage properties. However, structural in-situ observations have hitherto not been possible owed to the lack of crystallinity of such intermediates. The new series of compounds presented herein adds numerous new properties to the vast family of existing perovskite materials, from unprecedented structural behaviours dominated by weak interactions, denoted di-hydrogen contacts, known from concepts of molecular chemistry, to a variety of physical properties all attainable on the same host lattice. The chemistry of anion-mixing is expanded by the highly dynamic complex BH 4 , which hosts a number of unique features. In particular, hydride-specific effects, unattainable by crystal engineering with other anions, can enrich the spectrum of mechanisms leading to lattice distortions and instabilities via weak interactions, as manifested for instance in the generation of large superlattices of borohydride perovskites. Thus, alternative mechanisms to generate lattice distortions in perovskites independent on orbital effects are presented here. Various approaches have been explored recently to stabilize ferroelectric distortions without the need of d-p hybridization requiring empty d -orbitals or ns 2 lone pairs. For instance, A -site-driven ferroelectrics, such as geometric and hybrid improper ferroelectrics, generated by ordered layering schemes [27] , [28] , [29] or purely electrostatic schemes as in YMnO 3 (ref. 30 ). Both the di-hydrogen H ··· H contacts between BH 4 -ligands as well as the non-spherical shape of the anion are expected to be novel geometric tools for complex hydride perovskites to influence not only polarity by the anion-substitution BH 4 − ← X − but also by lattice instabilities in novel candidate ferroelectrics. While these hosts, on a structural level, merge the lattice-type-specific characteristics with new BH 4 -specific anion dynamics, they also constitute the first complex hydride series that can meet the requirements for genuine structure-property design. A large diversity in properties is therefore addressed herein, which in addition to applications in hydrogen storage spans solid-state phosphors, pressure sensors and, in future, possibly new electronic devices. Exceptionally complex superlattices may be created to increase the number of crystallographically distinct emission sites, for instance to target white luminescence. Another, potentially useful, physical property of borohydrides is the interaction of elements with ionizing radiation. For instance, both boron and hydrogen have very high neutron cross-sections, providing an excellent pre-requisite for luminescent lanthanide-based scintillators using borohydride perovskites, for instance as thermal neutron detection devices. The discovery of CsPb(BH 4 ) 3 contrasts the widely accepted semi-empirical relationship between the electronegativity and the stability of borohydrides [18] , [19] , suggesting that further disregarded electronegative elements from the periodic table may be incorporated into borohydride lattices. Borohydrides or borohydride-halides have till now not been explored regarding their electronic properties in the solid state. Electronic states generated by BH 4 − molecular orbitals and introduced into the Pb- X − bands may be a new tool to manipulate the band structure of plumbohalides. The presented series of perovskites also contains light-weight materials potentially interesting for hydrogen storage applications. The usage of ammonium NH 4 + as A -site cation allows stabilizing ammonium borohydride for the first time at RT. This describes an approach that is not restricted to perovskite-type borohydrides and the incorporation of NH 4 + may be generalized to search for new hydrogen-rich compounds. A major drawback of boron and nitrogen-based hydrogen storage systems [24] is the possible evolution of ammonia NH 3 and diborane B 2 H 6 , which both lead to the failure of fuel cells. Neither of them are observed during the hydrogen release of NH 4 Ca(BH 4 ) 3 . In conclusion, this communication presents a range of new perovskite-type materials along with detailed investigations of structure and properties providing progress towards rational material design in complex hydrides. Sample preparation All samples investigated in this study were prepared by mixing appropriate quantities of starting materials and ball milling in argon atmosphere in a planetary Fritsch Pulverisette 7. Milling was performed at 600 r.p.m. with 60 repetitions at 2 min each and a 5-min break between each repetition to avoid overheating of the sample. Starting materials were purchased from Sigma-Aldrich: (KBH 4 , LiBH 4 , Ca(BH 4 ) 2 , Mg(BH 4 ) 2 , KCl, KBr, KI, CaCl 2 , CaBr 2 , CaI 2 , NH 4 Cl, CH 3 NH 3 Cl, EuCl 2 , CeCl 3 ), Katchem Ltd. (RbBH 4 , CsBH 4 ) or, in the case of not being commercially available, produced as outlined below. Sr(BH 4 ) 2 was synthesized according to a previously reported procedure [31] . For the neutron powder diffraction (NPD) experiment, isotope-enriched K 11 BH 4 was purchased at Katchem Ltd. and subsequently deuterated at 400 °C and p (D 2 )=100 bar. Deuteration was achieved to 90%, as estimated by Raman spectra on the product and refined later on with NPD data. Ca( 11 BD 4 ) 2 was synthesized in house. Synthesis of homoleptic monometallic lanthanide-borohydrides Mn(BH 4 ) 2 and M (BH 4 ) 3 ( M =Y or Gd) were prepared from a metathesis reaction between MnCl 2 or M Cl 3 ( M =Y or Gd) and LiBH 4 in appropriate ratios. The reactants were ball milled (BM) separately in a Fritsch Pulverisette 6 planetary mill under inert conditions (argon atmosphere) in 80-ml tungsten carbide containers and balls (o.d. 6 mm). The sample-to-balls mass ratio was approximately 1:30 and a speed of 400 r.p.m. was selected while 5 min BM and 2 min pauses for 70 min (total BM time of 50 min) were applied. Subsequently, the reactants were added under vigorous stirring to a 2 M solution of dimethyl sulphide borane complex (S(CH 3 ) 2 BH 3 ) in toluene. The solution was kept for 72 h at RT. S(CH 3 ) 2 BH 3 was filtered away leaving a solid mixture of M (BH 4 ) 3 ( M =Y or Gd) and LiCl. LiCl was removed from the samples by dissolution of Mn(BH 4 ) 2 or M (BH 4 ) 3 ( M =Y or Gd) in dimethyl sulphide (S(CH 3 ) 2 ). Samples were left in (S(CH 3 ) 2 ) for 24 h under vigorous stirring [32] . The solution was successively filtered to remove LiCl and concentrated in vacuo using a rotary evaporator at T =50 °C until all the excess dimethyl sulphide had been removed and a white/yellow solid remained. α -Y(BH 4 ) 3 and Gd(BH 4 ) 3 were obtained in an adduct-free form by applying dynamic vacuum and heating at T =140 °C for 3 h, whereas the Mn(BH 4 ) 2 was heated to 110 °C. Synchrotron and NPD Synchrotron radiation powder X-ray diffraction data were collected at the Swiss Norwegian Beamlines of the European Synchrotron Radiation Facility (ESRF, Grenoble, France), at beamline I11 of Diamond Light Source (Didcot, England), at the Materials Science Beamline of the Swiss Light Source (Paul Scherrer Institute, Villigen, Switzerland) and at the High Energy Materials Science Beamline of Petra III (Deutsches Elektronen-Synchrotron, Hamburg). The NPD experiment was performed at the instrument HRPT of SINQ (PSI). Wavelengths of the corresponding experiments were 0.82257, 0.82712, 0.82711, 0.2072 and 1.8857 Å, respectively. For X-ray diffraction, samples were loaded into 0.5-mm borosilicate capillaries; for neutrons, a double-walled vanadium container was used, containing 2.2 g of sample. The superstructure reflections were indexed and the corresponding structures solved in direct space using the software FOX [33] . After structure solution, the respective models were refined with TOPAS [34] . Structure determination of KCa(BH 4 ) 3 The characteristic cubic perovskite peaks were quickly identified on temperature-ramps collected between 100 and 700 K on the two-dimensional Pilatus M2 detector of SNBL BM01A. Superstructure reflections for both low-temperature and high-temperature polymorphs show excellent statistics on 2D data. The high-temperature polymorph is better crystallized, this was indexed first to an orthorhombic cell related by (sqrt2/sqrt2/2) to a hypothetical cubic KCa(BH 4 ) 3 prototype. After detailed inspection, two choices of space group remained, related by inversion symmetry, Pnma in setting Pbnm and Pna 2 1 in setting Pbn 2 1 . The powder X-ray diffraction data did not allow to unambiguously determine the space group, but Rietveld refinements as well as sequential refinements turned out to be more stable for the non-centrosymmetric setting, Pbn 2 1 , which agrees well with the lower DFT energies ( Supplementary Table 2 ) for this model. Indexing of the low-temperature polymorph was much more challenging. In order to obtain the final model Pba 2 for bulk LT -KCa(BH 4 ) 3 , a full mode decompositions with Amplimodes [35] were performed to establish possible relations between different distortion modes in different parent symmetries. A full set of solid-state calculations on all models that made sense from a theoretical and diffraction point of view was also carried out. Supplementary Table 2 provides representative DFT optimizations showing fully relaxed converged models. Mode analysis Distortion modes in the different polymorphs of KCa(BH 4 ) 3 were analysed with the Amplimodes [35] applet available on the Bilbao crystallographic server ( http://www.cryst.ehu.es/ ), allowing to identify distortions that correspond to well-known soft modes frequently occurring in the perovskite lattice. The displacements were derived from the supposed tetragonal prototype P 4/ mbm that is approached before the structural phase transition. In polar Pba 2 and P 2 1 2 1 2, the polar mode causing displacement along the unique pseudotetragonal axis was discarded by shifting the origin so that Ca atoms come to lie on (0/0/0) in all different models. The tetragonal prototype itself of course is derived from a cubic Pm -3 m cell. To discuss the transition, however, it is useful to bring both orthorombic superstructures into context with P 4/ mbm . Rietveld refinements Structural refinements were carried out on all models allowing for the given lattice metric as derived above from the cubic prototype and compliant with crystallographic extinctions. BH 4 was modelled as a rigid body in TOPAS [34] with one free internal parameter being the bond length B-H. The same antibump restraints were applied in all refinement to ensure consistent refinements. For the case study on KCa(BH 4 ) 3 , the orientation of the BH 4 tetrahedron was additionally verified by refinements against neutron data collected at 15 K. Neutron data at high temperatures were not of sufficient quality to refine the high-temperature phase of KCa(BH 4 ) 3 . Vibrational spectroscopy Infrared spectra were collected on a Bio-Rad Excalibur instrument (Bio-Rad; spectral resolution of 1 cm −1 ) and Raman spectra with a 488-nm solid-state laser and a Kaiser optical Holospec monochromator equipped with a liquid-cooled CCD (charge-coupled device) camera. Thermogravimetric analysis Differential scanning calorimetry and thermogravimetry were performed with a Netzsch 404 F3 Pegasus apparatus (Netzsch) under nitrogen flow. Photophysical measurement RT emission and excitation spectra were obtained using a Fluorolog 3-22 instrument. Variable temperatures down to 10 K were achieved with a closed cycle cryosystem (Janis-Sumitomo SHI-4-5, Janis) equipped with a computer-controlled temperature controller. Photo-excitation was carried out using the third harmonics of the Nd:YAG-pulsed laser (355 nm, pulse energy around 1 mJ per pulse, 20 Hz). Luminescence spectra were measured using a 0.28 m monochromator (Spex 280 M) equipped with a CCD camera (Jobin-Yvon CCD 3500, 150 g mm −1 grating). Luminescence kinetics were measured using the home-built 0.28 m monochromator (Spex 280 M) equipped with a photo multiplier (PM) tube. Absorption spectra were collected on a Bruker 66 FT-IR setup (Bruker). Computational details All the solid-state calculations were performed at DFT level of theory using the Vienna Ab initio Simulation Package ( VASP ) code [36] , [37] , [38] . A hybrid PBE0 functional [39] was used to optimize the structures. Plane waves formed a basis set and the calculations were performed using the projector-augmented wave method [40] , [41] and atomic pseudo-potentials [42] . The energy cutoff controlling the accuracy of calculations was set to 1,000 eV. Brillouin zones were sampled during structure optimization in 4/8 (DFT/Hartree-Fock) and in 32/64 (DOS calculation) k -points, respectively [43] , [44] . The positions of all the atoms in the respective computational cells were fully relaxed with both the lattice vectors fixed and optimized. Trajectories between special points of respective Brillouin zones were sampled in 10 k -points. How to cite this article: Schouwink, P. et al. Structure and properties of complex hydride perovskite materials. Nat. Commun. 5:5706 doi: 10.1038/ncomms6706 (2014).